Analysing the substrate multispecificity of a proton-coupled oligopeptide transporter using a dipeptide library Peptide uptake systems that involve members of the proton-coupled oligopeptide transporter (POT) family are conserved across all organisms. POT proteins have characteristic substrate multispecificity, with which one transporter can recognize as many as 8,400 types of di/tripeptides and certain peptide-like drugs. Here we characterize the substrate multispecificity of Ptr2p, a major peptide transporter of Saccharomyces cerevisiae , using a dipeptide library. The affinities ( K i ) of di/tripeptides toward Ptr2p show a wide distribution range from 48 mM to 0.020 mM. This substrate multispecificity indicates that POT family members have an important role in the preferential uptake of vital amino acids. In addition, we successfully establish high performance ligand affinity prediction models (97% accuracy) using our comprehensive dipeptide screening data in conjunction with simple property indices for describing ligand molecules. Our results provide an important clue to the development of highly absorbable peptides and their derivatives including peptide-like drugs. Peptide uptake systems are conserved across all organisms from bacteria to higher animals and plants and are important for acquiring nitrogen resources with high efficiency [1] , [2] , [3] , [4] , [5] , [6] . The molecules involved in these systems belong to the proton-coupled oligopeptide transporter (POT) family, which is also called the peptide transporter (PTR) family [3] . POT family members comprise 12 transmembrane domains as a general structure and have characteristic substrate multispecificity, by which one transporter can recognize a variety of substrates [7] . In humans, hPEPT1 expressed in the small intestine epithelium is involved in absorbing nutritional peptides [8] , [9] , [10] , whereas hPEPT2 expressed in the renal tubules is involved in the reabsorption of peptides from primitive urine [11] , [12] , [13] . Due to their substrate multispecificity, it is assumed that each of these POT family transporters can recognize as many as 8,400 types of di/tripeptides, which are products generated by protein hydrolysis, at a single substrate-binding site that resides on each transporter and can actively transport these peptides [7] , [14] , [15] . Furthermore, hPEPT1 and hPEPT2 can transport peptide-like drugs such as β-lactam antibiotics, anti-hypertensive drugs and anti-cancer agents [16] . This property influences the intestinal absorption of drugs and half-life of drugs in blood. For the yeast S. cerevisiae , Ptr2p is the major transporter involved in the uptake of di/tripeptides [17] , [18] , [19] , [20] . Because the uptake of amino acids in the peptide form is much faster than in the amino-acid form, peptide-based media can improve the growth of yeasts [6] , [21] . Although Ptr2p is an important protein for the fermentation industry, there is little information on the substrate preferences of Ptr2p [22] . As with the examples above, the substrate multispecificity of a POT family protein is of interest in various fields of science including drug development, nutrition and fermentation. The question of how one substrate-binding site can recognize a variety of substrates is the major focus in peptide transport research. To date, the necessary or important structural characteristics for recognition by POT family transporters have been proposed by determining the affinity of individual substrates for these transporters [23] , [24] , [25] . However, the entire spectrum of the substrate preference of POT family transporter has not been elucidated. In addition, the crystal structures of two bacterial POT family transporters, PepTso [14] from Shewanella oneidensis and PepTst [15] from Streptococcus thermophilus , were recently determined, which provided important clues for elucidating the substrate multispecificity of the POT family. Because the amino-acid sequence of PepTso is highly homologous to those of hPEPT1 and hPEPT2, PepTso is the best structural model currently available for these eukaryotic peptide transporters. The crystal structure of PepTso provided basic information on the three dimensional configuration of the amino-acid residues at its substrate-binding site. To advance further in designing a detailed pharmacophore map, it is necessary to elucidate the physicochemical characteristics that determine the affinity of a substrate for a POT family transporter. This study reports the substrate multispecificity of S. cerevisiae Ptr2p used as a model POT family transporter. Detailed substrate multispecificity of the Ptr2p was characterized by a comprehensive analysis using a dipeptide library and a high-throughput assay system developed by us. By constructing models to predict the dipeptide affinities for Ptr2p, we observed that ligand affinity K i values could be predicted in silico with high accuracy. For in silico model construction, we used a combination of simple ligand property parameters rather than using complex structural information for ligands and receptors. The biological mechanisms and roles of POT family proteins are discussed on the basis of careful examination of the prediction models constructed using different property parameters as descriptive parameters for ligand affinity. Construction of a Ptr2p expression system To avoid the activity of its endogenous peptide transporter, a PTR2 gene knockout strain ( S. cerevisiae BY4742- ptr2Δ ) was used as the host strain for Ptr2p expression (SC-Ptr2p). The membrane fraction of SC-Ptr2p cells was analysed by western blot using an anti-FLAG antibody to verify Ptr2p expression ( Fig. 1a ). Ptr2p was detected as a single band of 68 kDa, which was consistent with the size of the intact Ptr2p [19] . The FLAG tag was replaced with GFP at the carboxy terminus of Ptr2p and localization of the Ptr2p–GFP fusion protein was analysed by confocal fluorescence microscopy ( Fig. 1b ). The result indicated that Ptr2p–GFP was localized on the cell surface. Dipeptide uptake ability of SC-Ptr2p cells was then analysed ( Fig. 1c ). Strain BY4742 requires leucine and histidine in its growth medium. Thus, these amino acids were added to the growth medium in the form of dipeptides (His and Leu). SC-Ptr2p cells grew and formed colonies on these plates after absorbing these peptides, whereas its host strain did not grow. These results indicated that Ptr2p was potent, expressed exogenously and localized on the cell surface. 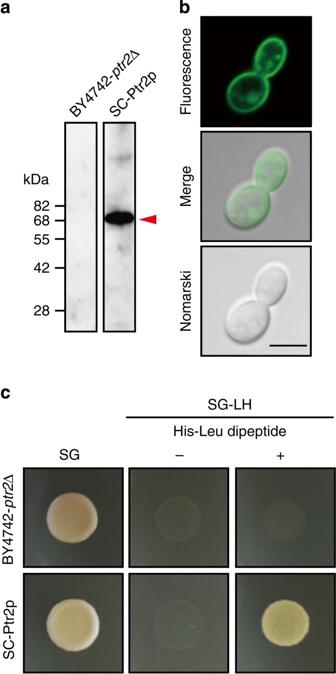Figure 1: Generation of Ptr2p-expressing cells. (a) Western blot analysis of the membrane fraction prepared from SC-Ptr2p cells (BY4742-ptr2Δ cells that expressed plasmid-borne Ptr2p) using an anti-FLAG antibody. Arrowhead indicates expressed Ptr2p. (b) Localization of a Ptr2p–GFP fusion protein using confocal fluorescence microscopy in BY4742-ptr2Δ. Scale bar represents 5 μm. (c) Spot assay. Dipeptide uptake capability of SC-Ptr2p cells was analysed. Leucine and histidine, which are required for the growth of strain BY4742 were added to the medium in the form of a dipeptide (His–Leu, 10 mM). Figure 1: Generation of Ptr2p-expressing cells. ( a ) Western blot analysis of the membrane fraction prepared from SC-Ptr2p cells (BY4742- ptr2 Δ cells that expressed plasmid-borne Ptr2p) using an anti-FLAG antibody. Arrowhead indicates expressed Ptr2p. ( b ) Localization of a Ptr2p–GFP fusion protein using confocal fluorescence microscopy in BY4742- ptr2 Δ. Scale bar represents 5 μm. ( c ) Spot assay. Dipeptide uptake capability of SC-Ptr2p cells was analysed. Leucine and histidine, which are required for the growth of strain BY4742 were added to the medium in the form of a dipeptide (His–Leu, 10 mM). Full size image A fluorescence-based competitive uptake assay system A fluorescence-based competitive uptake (F-CUp) assay system is a high-throughput assay that determines the competitive-inhibitory activity (IC 50 ) of an analysed substrate versus the uptake of a tracer substrate. An IC 50 value can be converted to a K i value using the Cheng–Prusoff equation [26] . Functional analysis of Ptr2p was conducted using β-Ala–Lys (AMCA) as the tracer substrate to establish an F-CUp assay system. β-Ala–Lys (AMCA) uptake was mediated by Ptr2p and it accumulated within the vacuoles ( Fig. 2a ). This uptake was inhibited by the imidazole dipeptide carnosine as a representative result. The β-Ala–Lys (AMCA) uptake was time-dependent, and its uptake by the host strain was negligible ( Fig. 2b ). In previous experiments, it was demonstrated that most of the di/tripeptides were transported via Ptr2p in S. cerevisiae [6] . Thus, Ptr2p was a major transporter for both the tracer (β-Ala–Lys(AMCA)) and dipeptides. Furthermore, β-Ala–Lys (AMCA) uptake was also concentration dependent, and the K m value was calculated to be 0.16 (±0.02, s.d.) mM according to the Michaelis–Menten formula ( Fig. 2c ). The competitive-inhibitory activity was analysed using amino acids and oligopeptides with different chain lengths ( Fig. 2d ). Only di/tripeptides showed competitive-inhibitory effects against the uptake of the tracer substrate. The K i values for Gly–Gly and Gly–Gly–Gly were calculated to be 17 and 48 mM, respectively. To investigate whether differences in amino-acid sequences affected the affinity for Ptr2p, three different dipeptides, Ala–Ala, Ala–Leu and Leu–Ala, were analysed ( Fig. 2e ). The affinities of the two dipeptides that included leucine, Leu–Ala ( K i =0.15 mM) and Ala–Leu ( K i =0.31 mM), were higher than that of Ala–Ala ( K i =0.40 mM). The affinity of Leu–Ala was twice that of Ala–Leu. Thus, this demonstrated that in addition to the amino-acid composition, the amino-acid sequence also contributed to the affinity for Ptr2p. 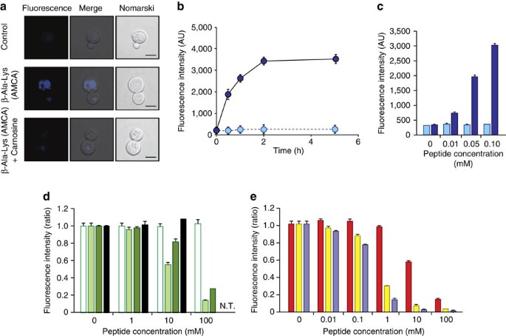Figure 2: Establishing the F-CUp assay system. (a) Analysis of tracer substrate, β-Ala–Lys (AMCA), uptake by SC-Ptr2p cells (BY4742-ptr2Δ cells that expressed plasmid-borne Ptr2p) using confocal fluorescence microscopy. Scale bar represents 5 μm. (b) Time course for the uptake of the tracer substrate (50 μM) in SC-Ptr2p. Dark blue: SC-Ptr2p cells, Light blue: parental strain BY4742-ptr2Δ. (c) Concentration dependence of tracer substrate uptake in SC-Ptr2p. Dark blue column: SC-Ptr2p cells; light blue column: parental strain BY4742-ptr2Δ cells. (d) Effect of peptide chain length on tracer substrate uptake based on competitive inhibition. White column: Gly; light green column: Gly–Gly, green column: Gly–Gly–Gly; dark green column: Gly–Gly–Gly–Gly. N.T.: not tested. (e) Effect of amino-acid sequence on tracer substrate uptake based on competitive inhibition. Red column: Ala–Ala, yellow column: Ala–Leu, purple column: Leu–Ala. Results of panelsb–eare means±s.d. (n=3). Figure 2: Establishing the F-CUp assay system. ( a ) Analysis of tracer substrate, β-Ala–Lys (AMCA), uptake by SC-Ptr2p cells (BY4742- ptr2 Δ cells that expressed plasmid-borne Ptr2p) using confocal fluorescence microscopy. Scale bar represents 5 μm. ( b ) Time course for the uptake of the tracer substrate (50 μM) in SC-Ptr2p. Dark blue: SC-Ptr2p cells, Light blue: parental strain BY4742- ptr2 Δ. ( c ) Concentration dependence of tracer substrate uptake in SC-Ptr2p. Dark blue column: SC-Ptr2p cells; light blue column: parental strain BY4742- ptr2 Δ cells. ( d ) Effect of peptide chain length on tracer substrate uptake based on competitive inhibition. White column: Gly; light green column: Gly–Gly, green column: Gly–Gly–Gly; dark green column: Gly–Gly–Gly–Gly. N.T. : not tested. ( e ) Effect of amino-acid sequence on tracer substrate uptake based on competitive inhibition. Red column: Ala–Ala, yellow column: Ala–Leu, purple column: Leu–Ala. Results of panels b – e are means±s.d. ( n =3). Full size image Relationship between Ptr2p affinity and S. cerevisiae growth The affinity of dipeptides for Ptr2p and their effects on the growth of S. cerevisiae were examined using two different combinations of dipeptides: His–Leu and Leu-His or Leu-Gly and Gly-Leu ( Fig. 3 ). The K i values of His–Leu, Leu-His, Leu-Gly and Gly-Leu were 0.05, 0.13, 0.36 and 0.60 mM, respectively. Yeast cell growth analysis indicated that those dipeptides with lower K i values were better nutrients for Ptr2p-expressing yeast despite their identities in terms of their amino-acid composition. The effect for improving cell growth by a high-affinity peptide was also verified using the FGY217 strain, which did not artificially express Ptr2p ( Supplementary Fig. S1 ). The F-CUp assay system combined with growth analysis can also be a useful tool for developing an efficient fermentation medium. 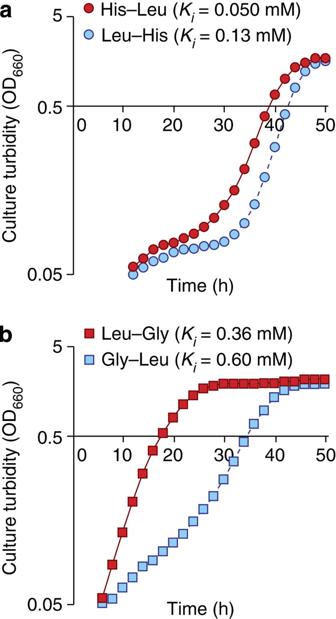Figure 3:Relationship between affinity for Ptr2p andS. cerevisiaegrowth. Analysis using dipeptides (a) comprising histidine and leucine (b) comprising glycine and leucine. Pre-cultures of the BY4742 strain were diluted to give OD660=0.06 in each test medium (10 mM of each dipeptide, 0.14% yeast synthetic drop-out medium without leucine, 0.67% yeast nitrogen base without amino acids and 2% galactose) and incubated at 30 °C. Figure 3: Relationship between affinity for Ptr2p and S. cerevisiae growth. Analysis using dipeptides ( a ) comprising histidine and leucine ( b ) comprising glycine and leucine. Pre-cultures of the BY4742 strain were diluted to give OD 660 =0.06 in each test medium (10 mM of each dipeptide, 0.14% yeast synthetic drop-out medium without leucine, 0.67% yeast nitrogen base without amino acids and 2% galactose) and incubated at 30 °C. Full size image F-CUp assay using a dipeptide library We performed a comprehensive analysis using a dipeptide library by the F-CUp assay system to characterize the substrate multispecificity of Ptr2p ( Fig. 4a ). For 338 types of dipeptides that could be synthesized, we calculated the K i values of 237. K i values could not be calculated for substrates for which the IC 50 values were above 1.0 mM due to their poor solubility. Instead, their K i values were assigned to be greater than 0.77 mM. 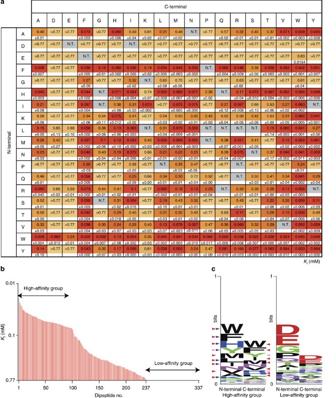Figure 4: Substrate multispecificity of Ptr2p. (a) Comprehensive analysis using a dipeptide library by the F-CUp assay system. Colours of cells correspond toKivalues. N.T.: not tested. Data are presented as means±s.d. (n=3). (b) Distribution ofKivalues. (c) Frequency analysis of amino-acid residues with high or low-affinity dipeptides using the WebLogo programme (http://weblogo.berkeley.edu/). Blue, red and pink arrowheads indicate N-end rule amino acids in yeast, essential amino acids and semi-essential amino acids for humans, respectively. Figure 4: Substrate multispecificity of Ptr2p. ( a ) Comprehensive analysis using a dipeptide library by the F-CUp assay system. Colours of cells correspond to K i values. N.T. : not tested. Data are presented as means±s.d. ( n =3). ( b ) Distribution of K i values. ( c ) Frequency analysis of amino-acid residues with high or low-affinity dipeptides using the WebLogo programme ( http://weblogo.berkeley.edu/ ). Blue, red and pink arrowheads indicate N-end rule amino acids in yeast, essential amino acids and semi-essential amino acids for humans, respectively. Full size image The calculated K i values showed a wide range distribution ( Fig. 4b ). Trp-Phe exhibited the highest affinity ( K i =0.020 mM). It was also found that their affinities for Ptr2p were 2,400 times higher than those with the lowest affinity: Gly–Gly–Gly with K i =48 mM analysed in this study. We selected a group of high-affinity dipeptides with K i values below 0.077 mM and a group of low-affinity dipeptides with K i values above 0.77 mM. We used these in an appearance frequency analysis of the amino-acid residues using the WebLogo programme ( Fig. 4c ). This showed that dipeptides containing aromatic amino acids (namely Phe, Trp and Tyr) and branched-chain amino acids (namely Ile, Leu and Val) frequently appeared in the high-affinity group. On comparing, it was found that the low-affinity group had a high frequency of negatively charged amino acids (that is, Asp and Glu), as well as amino acids that were predicted to influence peptide bond conformation (that is, Gly and Pro). In both groups of dipeptides, amino-acid residues at the amino terminus showed a higher propensity compared with those at the C-termini, which suggested that an amino-acid residue at the N-terminus had a more significant role in recognition by Ptr2p than those in the C-terminus. Constructing ligand affinity prediction models To expand the applications of our assay data, we constructed discrimination analysis models to predict ligand affinity in silico ( Table 1 ). Our assay data comprised discrete over-threshold data ( K i >0.77) for several low-affinity dipeptides within continuous K i data, along with future screening applications for in silico pre-screening; therefore, we selected discrimination analysis models to predict categorical labels for ligand molecules. Compared with conventional ligand prediction models, we selected features that could be simply calculated from the primary sequences of dipeptides as descriptive parameters to construct simple prediction models that utilizes fewer parameters. Table 1 Prediction results of dipeptide affinity discrimination models with their parameter selection processes. Full size table We examined a total of six prediction models and observed that categorizing dipeptide samples as high, medium or low can predict affinities with extremely high accuracy (average prediction>84%). By comparing the data set type for whether or not it included intermediate K i ligands, we observed that 97% prediction accuracy (data set type B, prediction model type M2) can be achieved for objectively screening ligands that would interact with Ptr2p. Even with data set type A modelled by M2, predictions were accurate in the area of ‘extremely high-affinity samples’, which indicated sufficient applicability for ligand screening ( Supplementary Fig. S2 ). By comparing these prediction model types, we observed that the combined information on amino-acid residues and chemical property information was most effective for obtaining an accurate prediction model. Prediction accuracy slightly increased by adding chemical property parameters that described total ligand molecular properties. However, sufficient prediction accuracy was achieved by converting the primary sequences of dipeptides into a few amino-acid indices. In addition, we observed that even without amino-acid information, total molecular chemical property information could be used as an alternative parameter to maintain similar prediction accuracy. From the parameter selection process of constructing six discrimination analysis models, the manner of a dipeptide–Ptr2p interaction could be determined. During the modelling process with model M1, index 3 (side-chain contribution to protein stability) at the N-terminal, index 14 (side-chain interaction parameter) and indices 8 and 1 (isoelectric point) were the first four parameters that greatly contributed to the increased prediction accuracy. These results were common physicochemical rules for interactions between dipeptides and Ptr2p, which could be extracted from our comprehensive dipeptide library assay data. This extraction rule by model analysis was only possible with the affinity data with variety, and would not be attainable from partial positive screening data obtained from conventional, limited size assays. In addition to the discriminant analysis models that predicted the categories of ligand affinities, multiple regression models that predicted K i values directly from molecular properties were observed to provide sufficient accuracy for screening (corrected R 2 values>0.734). PTR2 gene expression controlled by an N-end rule dipeptide To examine the effect of amino-acid sequence of dipeptide on PTR2 gene expression, we analysed yeasts grown in YPD media containing dipeptides Ala–Ala or Trp–Ala ( Fig. 5 ). In a direct analysis of gene expression by the FGY217 strain using real time RT–PCR, PTR2 gene expression increased twofold by adding the N-end rule dipeptide Trp–Ala in the YPD medium as compared with adding the non N-end rule dipeptide Ala–Ala. 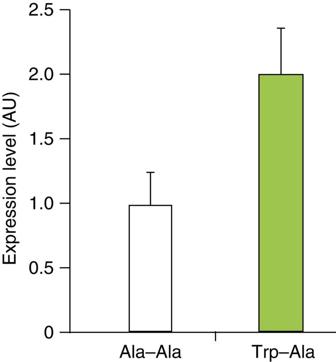Figure 5:PTR2gene expression controlled by an N-end rule dipeptide. Pre-cultures of the FGY217 strain were diluted to give OD660=0.06 in each test YPD medium (2% peptone, 1% yeast extract, 2% glucose and 10 mM Trp–Ala or Ala–Ala), and then grown at 30 °C for 5 h.PTR2gene expression was analysed by real time RT–PCR. Data are presented as means±s.d. (n=3). Figure 5: PTR2 gene expression controlled by an N-end rule dipeptide. Pre-cultures of the FGY217 strain were diluted to give OD 660 =0.06 in each test YPD medium (2% peptone, 1% yeast extract, 2% glucose and 10 mM Trp–Ala or Ala–Ala), and then grown at 30 °C for 5 h. PTR2 gene expression was analysed by real time RT–PCR. Data are presented as means±s.d. ( n =3). Full size image In this study, the substrate multispecificity of Ptr2p, the major peptide transporter of S. cerevisiae , was characterized using an F-CUp assay system ( Fig. 4 ). Although there have been several reports regarding affinity analyses of substrates for POT family members [7] , [27] , [28] , [29] , this is the first study to use a dipeptide library for a comprehensive analysis. From this library assay data, we also successfully constructed in silico ligand affinity prediction models for Ptr2p using discriminant analysis models. By analysing the model construction processes, new insights were obtained to further understand the manner of interactions between dipeptides and Ptr2p. The primary structure of Ptr2p was compared with that of other family members to gain a better understanding of the substrate recognition mechanism of a POT family protein. Although the similarity between the primary structure of Ptr2p and that of PepTso was 33.7% ( Supplementary Fig. S3 ), three dimensional structures suggested that 12 amino-acid residues comprising the substrate-binding site of PepTso were highly conserved among these family members ( Fig. 6a ). For Ptr2p, 11 amino-acid residues, excluding Ser100 (corresponds to Arg32 in PepTso)( Supplementary Fig. S3 ), were functionally similar to those of PepTso. Dipeptides that comprise aromatic amino acids displayed high affinity for Ptr2p, whereas dipeptides that comprise negatively charged amino acids displayed low affinity for Ptr2p ( Fig. 4c ). The results obtained using individual substrates indicated that the substrate preferences of hPEPT1, hPEPT2, PepTst and YjdL were similar to those of Ptr2p ( Fig. 6b ) [7] , [15] , [30] . This consistency likely indicates that POT family members share a common substrate recognition mechanism. This was supported by the fact that the substrate-binding sites of these family members comprise highly conserved amino-acid residues. 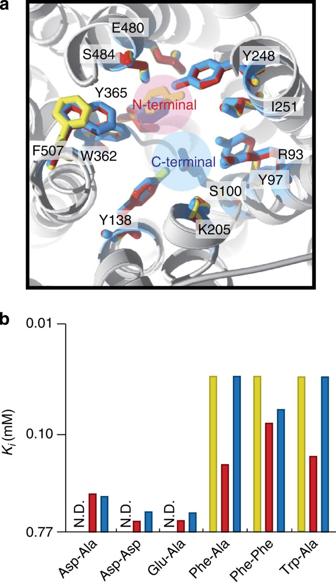Figure 6: Substrate recognition shared among POT family members. (a) Close view of the substrate-binding site structures. Homology models for Ptr2p and hPEPT1 were constructed using the SWISS-MODEL programme (http://swissmodel.expasy.org/) with PepTso (PDB: 2XUT) as a template14. Structures of Ptr2p and hPEPT1 are superimposed on the PepTso structure. The PepTso structure is shown as a ribbon model and the amino-acid residues that interact with a substrate peptide in PepTso are shown as a stick model. Blue: PepTso, yellow: Ptr2p, red: hPEPT1. Putative binding substrates are shown as pink and blue circles. (b) Dipeptide affinity for each transporter.Kivalues for hPEPT1 and hPEPT2 are from published data7. ND: not determined (Ki>0.77 mM). Yellow column: Ptr2p, red column: hPEPT1, blue column: hPEPT2. Figure 6: Substrate recognition shared among POT family members. ( a ) Close view of the substrate-binding site structures. Homology models for Ptr2p and hPEPT1 were constructed using the SWISS-MODEL programme ( http://swissmodel.expasy.org/ ) with PepTso (PDB: 2XUT) as a template [14] . Structures of Ptr2p and hPEPT1 are superimposed on the PepTso structure. The PepTso structure is shown as a ribbon model and the amino-acid residues that interact with a substrate peptide in PepTso are shown as a stick model. Blue: PepTso, yellow: Ptr2p, red: hPEPT1. Putative binding substrates are shown as pink and blue circles. ( b ) Dipeptide affinity for each transporter. K i values for hPEPT1 and hPEPT2 are from published data [7] . ND: not determined ( K i >0.77 mM). Yellow column: Ptr2p, red column: hPEPT1, blue column: hPEPT2. Full size image In S. cerevisiae , Ptr2p expression is regulated by the N-end rule pathway [31] , [32] , [33] , by which the binding of dipeptides with a certain N-terminus to Ubr1p promotes the degradation of Cup9p, which is a repressor of the PTR2 gene. Thus, the Ptr2p expression level increases when peptides that meet the N-end rule are imported. Cai et al. [22] reported that several N-end rule peptides were preferentially recognized by Ptr2p. This is consistent with our present results obtained from a comprehensive analysis of a dipeptide library. The N-terminus of our high-affinity group is consistent with amino acids that adhered to the N-end rule (Trp, Phe, His, Tyr, Leu, Ile and Lys; Fig. 4c ). Interestingly, most of the essential and semi-essential amino acids for humans (Trp, Phe, His, Tyr, Met, Leu, Ile, Val, Lys and Arg) were also the constituent amino acids of high-affinity peptides ( Fig. 4c ). In general, the biosynthesis of aromatic amino acids requires the expression of multiple enzymes and involves energy-consuming reactions, whereas biosynthesis of acidic amino acids occurs from shorter branches of the TCA cycle [34] . The substrate multispecificity of the POT family of transporter, revealed by analysing Ptr2p, indicates that these family members are involved in the preferential uptake of specific amino acids that impose a biosynthesis burden on organisms ( Fig. 4c ). Based on this perspective, we propose the following positive feedback model for peptide uptake into S. cerevisiae ( Fig. 7 ). (i) Peptides with vital amino acids are preferentially transported into S. cerevisiae cells based on the substrate multispecificity of Ptr2p. (ii) Peptide uptake is accurately sensed by the N-end rule pathway via Ubr1p. (iii) Subsequently, Ptr2p expression is promoted after Cup9p degradation. (iv) S. cerevisiae cells can then more efficiently absorb those vital amino acids in their peptide form. Enhanced PTR2 gene expression by a transported dipeptide was experimentally demonstrated using an N-end rule dipeptide, Trp–Ala ( Fig. 5 ). The association between the substrate multispecificity of Ptr2p and the regulatory system for PTR 2 gene expression is biologically reasonable. 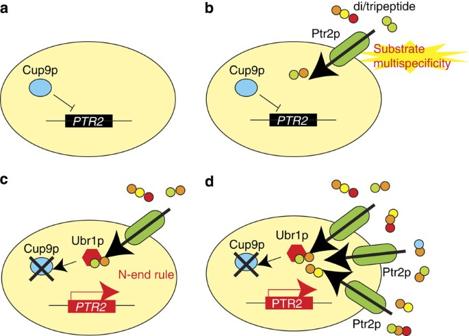Figure 7:Positive feedback model for peptide uptake intoS. cerevisiae. (a)PTR2gene expression is repressed by Cup9p. (b) Peptides with vital amino acids are preferentially transported into yeast cells based on the substrate multispecificity of Ptr2p. (c) Peptide uptake is accurately sensed by the N-end rule pathway via Ubr1p, following which Ptr2p expression is further promoted after Cup9p degradation31,32,33. (d)S. cerevisiaecells can then more efficiently absorb these vital amino acids in their peptide form. Figure 7: Positive feedback model for peptide uptake into S. cerevisiae . ( a ) PTR2 gene expression is repressed by Cup9p. ( b ) Peptides with vital amino acids are preferentially transported into yeast cells based on the substrate multispecificity of Ptr2p. ( c ) Peptide uptake is accurately sensed by the N-end rule pathway via Ubr1p, following which Ptr2p expression is further promoted after Cup9p degradation [31] , [32] , [33] . ( d ) S. cerevisiae cells can then more efficiently absorb these vital amino acids in their peptide form. Full size image By examining our prediction models, we observed that a few simple parameters that could be obtained from ligand sequence information could produce high accuracy ligand prediction models. The accuracy and the construction processes indicated that a few physicochemical properties of dipeptides were sufficient for discriminating their affinities for Ptr2p. Our prediction model accuracy strongly suggests that Ptr2p recognition is primarily governed by ‘property combinations’ that characterize the physiochemical properties of ligands rather than their exact sequence motifs. By comparing different types of descriptive parameters that can be derived from the same dipeptide sequence (M1, M2 and M3 comparisons in Table 1 ), we observed that the best prediction accuracy can be obtained when both ‘amino-acid-specific physicochemical properties’ and ‘total molecular chemical property’ were used as descriptors for dipeptide molecules. However, similar affinity prediction accuracy for Ptr2p was retained even after eliminating the ‘amino acid-specific physicochemical properties’. These results indicate that our affinity prediction models constructed in silico are applicable to pre-screening for medical applications. To examine this possibility, we compared the experimental and predicted binding affinities to Ptr2p for six medical compounds as a trial ( Supplementary Table S1 ). The predicted results matched F-CUp assay results for alafosfalin, arphamenine B, valacyclovir and captopril, although they did not match for fosinopril and benazepril. Based on the distribution of their molecular sizes, we assumed that the constructed prediction model using dipeptide library affinity data could predict the affinities for molecules that were close in size to those of dipeptides, having an average molecular weight of 256. In other words, it was reasonable that the predicted performance was limited to the variations of the ‘molecular chemical properties’ that existed in the dipeptide library used for model training. Therefore, increasing the ‘molecular information’ to train for wider variations in transporter affinities along with adding descriptive parameters will be the focus of our next investigation to expand our prediction approach. However, despite its limited application, it should be noted that our F-CUp assay-derived exhaustive molecular interaction data together with this modelling concept has great potential for affinity predictions of dipeptide-like molecules with high accuracy. Compared to the transported prediction approaches demonstrated by Biegel et al. [25] , our affinity prediction approach is sufficient for affinity predictions using only simple and feasibly calculated parameters for molecules without any prior ligand structural information. The model construction process also guided our understanding of dipeptide interactions with Ptr2p. In M1 models ( Table 1 ), index 3 (side-chain contribution to protein stability) at the N-terminal, index 14 (side-chain interaction parameter) and indices 8 and 1 (isoelectric point) were reproducibly selected in the same order in two models using data set type A or B. Index 3 and index 14 are strongly related to residues with ‘aromatic rings’ and ‘interactive residues’ that can stabilize molecular interactions ( Supplementary Table S2 ). Indices 8 and 1 and some parts of index 14 can be interpreted as ‘effect of charged and polarized residues’. Therefore, these two physicochemical property features can be considered as the main determining factors for Ptr2p ligand recognition. Several substrate characteristics for binding have been elucidated based on the interaction data for many ligands with POT family transporters. For PEPT1, binding models were proposed by Foley et al. , Brandsch et al. , and Daniel and Kottra [23] , [35] , [36] . According to these models, the properties of the individual residues at both the N- and C-termini are important. While the interactions between a peptide backbone, side-chains and the binding pocket are not completely understood, all of these models indicate that a bulky, hydrophobic side chain is advantageous for high affinity towards PEPT1. On comparing, acidic amino acids in the N-terminus resulted in a greater reduction in affinity than did the same amino acids in the C-terminus. These models for PEPT1 are consistent with our results based on an in silico analysis of Ptr2p in nature. Therefore, from a general point of view, this also supports the hypothesis that POT family members share a common substrate recognition mechanism. Most organisms, including yeasts and humans, have both peptide transporters and amino-acid transporters and both types of transporters cooperatively contribute to amino-acid resource uptake. The rates of substrate uptake by peptide transporters are higher than those of amino-acid transporters [4] , [5] , [6] . Therefore, an important role of peptide transporters is to import amino acids that are found in bulk in the extracellular fluid with high efficiency. To perform this role, peptide transporters must have substrate multispecificity in order to recognize a variety of compounds. Ligand recognition by hydrophobic interactions as well as by π−π bonds, which are not strictly directional, is suitable for this purpose. It is likely that POT family proteins have evolved so that these transporters have become equipped with such a substrate recognition mechanism ( Table 1 ). The fact that many of the amino-acid residues that are involved in substrate binding are aromatic amino acids supports these characteristics ( Fig. 6 ) [14] , [15] . An ‘ambiguous’ substrate recognition mechanism, which is primarily based on physicochemical properties with no strict directionality, is the basis for substrate multispecificity and causes POT family members to act as drug transporters to absorb drugs, which are not natural substrates [37] , [38] , [39] . This ‘ambiguous’ substrate recognition mechanism was also observed in our regression analysis. The concept of affinity prediction for POT family members using combinations of amino-acid indices has a great potential to be extended to other targets for predicting the affinities of as many as 8,000 tripeptides [40] . The concept of using combinations of physicochemical properties for affinity prediction can also be applied to the information of structural properties used in structure-based drug design, which is becoming possible owing to the elucidation of the crystal structures of POT family members [14] , [15] . Therefore, the analytical data from this research provides important information for detailed pharmacophore mapping. Materials and chemicals β-Ala–Lys (AMCA) was purchased from Biotrend (Cologne, Germany). Substrate dipeptides were purchased from Anaspec (California, USA). The S. cerevisiae strains BY4742 ( MAT α , his3Δ1, leu2Δ0, lys2Δ0, ura3Δ0 ) and BY4742- ptr2Δ were purchased from Open Biosystems (Alabama, USA). Preparation of Ptr2p-expressing cells (SC-Ptr2p) PCR was used to isolate the PTR2 gene from the genome of S. cerevisiae FGY217 ( MATa, ura3-52, lys2Δ201, pep4Δ ). The gene-specific primers 5′- ACCCCGGATTCTAGAACTAGTGGATCCCCC ATGCTCAACCATCCCAGCCAAG -3′ and 5′- AAATTGACCTTGAAAATATAAATTTTCCCC TCACTTGTCATCGTCGTCCTTGTAGTC ATATTTGGTGGTGGATCTTAGAC -3′ were used to obtain PCR fragments of the PTR2 gene. These primers contained gene-specific regions (bold) and homologous regions (Italic). A PCR fragment and the SmaI -linearized pRS426 GAL1 vector were co-transformed into BY4742- ptr2Δ cells. These two DNAs were then linked via homologous recombination [41] , [42] , [43] . Cells were spread on a selection plate (2% agar, 0.2% yeast synthetic drop-out medium without uracil, 0.67% yeast nitrogen base without amino acids and 2% glucose). Transformants were cultured at 30 °C for 48 h. The resulting transformants were Ptr2p-expressing cells: SC-Ptr2p. For the expression of Ptr2p, SC-Ptr2p cells were grown in selection medium (0.2% yeast synthetic drop-out medium without uracil, 0.67% yeast nitrogen base without amino acids and 2% glucose). After pre-culture at 30 °C for 24 h, cells were diluted to give an OD 660 =0.06 in induction medium (0.2% yeast synthetic drop-out medium without uracil, 0.67% yeast nitrogen base without amino acids and 2% galactose) cultured at 30 °C for 24 h. Confocal microscopy To express the Ptr2p–GFP fusion protein, 5′- AAATTGACCTTGAAAATATAAATTTTCCCC ATATTTGGTGGTGGATCTTAGAC -3′ was used as a reverse primer. Expression of the Ptr2p–GFP fusion protein used the same method as for Ptr2p. The localization of the Ptr2p–GFP fusion protein was analysed by detecting GFP fluorescence using an LSM-700 (Carl Zeiss MicroImaging, New York, USA). Spot assay SC-Ptr2p cells were grown in pre-culture medium at 30 °C for 24 h. Cells were spotted on an assay plate (10 mM His–Leu dipeptide, 0.14% yeast synthetic dropout medium without histidine, leucine and uracil, 0.67% yeast nitrogen base without amino acids, 2% galactose and 2% agar) and cultured at 30 °C for 5 days. Fluorescence-based Competitive Uptake (F-CUp) assay After induction, SC-Ptr2p cells were harvested by centrifugation and re-suspended in F-CUp assay buffer (150 mM NaCl, 50 mM Na-phosphate buffer; pH 6.0). Cells were harvested by centrifugation and re-suspended in F-CUp assay buffer to OD 660 =15. Cells were incubated with 0.05 mM β-Ala–Lys (AMCA) as a tracer substrate and at arbitrary concentration for oligopeptide analysis at 30 °C for 60 min. β-Ala–Lys (AMCA) is a dipeptide containing a fluorophore. Cells were washed three times with the F-CUp assay buffer. β-Ala–Lys (AMCA) uptake was quantified by whole-cell fluorescence (excitation at 355 nm and emission at 460 nm) using Flexstation III (Molecular Devices, California, USA). K m values were estimated using Lineweaver–Burk plot. The initial velocity of a reaction was determined from the fluorescence intensity increase during the first hour. At this point, the substrate concentration remained the same as the initial condition. The IC 50 value was estimated based on the reduced fluorescence by competitive inhibition of the tracer uptake. The K i value was calculated using the Cheng–Prusoff equation from the K m of β-Ala–Lys (AMCA) and the IC 50 of the analysed oligopeptide [26] . The mean K m value was used to calculate K i values. Thus, the error for estimating K m values was not included in the error when determining K i . This competition assay system can estimate the affinity of a substrate for a peptide transporter. Some dipeptides were actually transported by yeast cells based on their K i values for Ptr2p ( Fig. 3 ), although affinity does not always mean that a compound will be transported. Cell growth analysis For time course analysis of culture turbidity, strain BY4742 was grown overnight in culture medium (0.2% yeast synthetic medium, 0.67% yeast nitrogen base without amino acids and 2% glucose) at 30 °C for 24 h. Pre-cultures were diluted to give OD 660 =0.06 in each test medium (10 mM each dipeptide, 0.14% yeast synthetic dropout medium without leucine, 0.67% yeast nitrogen base without amino acids and 2% glucose) and incubated at 30 °C. Culture turbidity was monitored by measuring OD 660 using a Biophotorecorder TVS 062CA (Advantec, Tokyo, Japan). Ligand affinity prediction models and discrimination analysis Using the data set of dipeptide sequences in conjunction with their affinity data from the F-CUp assay, dipeptide affinity prediction models were constructed using discrimination analysis with PASW version 18, release 18.0.0 (IBM Corporation, Armonk, NY, USA). For objective variables (that is, teaching signals), experimentally determined K i values were grouped into three categories: low K i samples with K i <0.1, N =102; high K i samples with K i >0.77, N =100; and medium K i for the remaining samples, N =135. For predictor variables (that is, input parameters), dipeptide sequences were converted into two types of parameters. Type I parameters included seven amino-acid indices, which were calculated by converting each amino acid at either the N-terminal or the C-terminal side of dipeptides using amino-acid indices (AA index1, Genome Net Japan, organized by Kyoto University; http://www.genome.jp/dbget-bin/www_bfind?aaindex1 ) [44] . All indices in the database ( N =544, version 9.1, as of August 2006) were previously analysed by hierarchical clustering; seven indices [45] , [46] , [47] , [48] , [49] , [50] were chosen as independent indices that represented seven major independent clusters, which demonstrated no multicolinearity ( Supplementary Table S2 ). Type II parameters included 10 physicochemical property parameters, which were obtained from each total dipeptide molecule with an original pipeline protocol using Chemistry Component Collection in Pipeline Pilot (Accelrys, San Diego, CA, USA). For modelling, two different prediction concepts were compared with two types of data sets: type A data sets to construct prediction models to discriminate all three types of K i samples (high, medium and low); and type B data sets to construct prediction models to discriminate either low Ki samples or high K i samples. For both prediction concepts, three different prediction models were constructed: M1 prediction models using only type I parameters; M2 prediction models using type I and type II parameters and M3 prediction models using only type II parameters for comparing model performances between the different types of parameters. During the model construction process, a parameter increasing and decreasing method was employed with a threshold of P <0.20 based on F-Test for parameter selection. Model accuracy was evaluated based on the discrimination accuracy of either each teaching signal category or as a total. Real time RT–PCR A FGY217 strain pre-culture was diluted to give OD 660 =0.06 in each test YPD medium (2% peptone, 1% yeast extract, 2% glucose and 10 mM Trp–Ala or Ala–Ala), and then grown at 30 °C for 5 h. Yeast total RNA was isolated using a NucleoSpin RNA II kit (Machery-Nagel, Diiren, Germany) according to the manufacturer's protocol. The amount of total RNA was quantified by monitoring absorbance at 260 nm. The first strand was synthesized using a PrimeScript RT reagent kit (Takara, Shiga, Japan). Quantitative real time PCR analysis was done with a Thermal Cycler Dice Real Time System (Takara, Shiga, Japan) using SYBR Premix EX Taq (Takara, Shiga, Japan) and specific primers. The following gene-specific primers were used: 5′-CCACCATGTTCCCAGGTATT-3′ and 5′-CCAATCCAGACGGAGTACTT-3′ for ACT1 ; and 5′-CAGTGACCGTTGATCCTAAAT-3′ and 5′-CTGAAGCACAACCAGAACAAA-3′ for PTR2 . PTR2 mRNA levels were normalized to those of ACT1 values using the 2- ΔΔ CT method. We calculated the fold-change of PTR2 mRNA in YPD medium containing Trp–Ala compared to that containing Ala–Ala. How to cite this article: Ito, K. et al. Analysing the substrate multispecificity of a proton-coupled oligopeptide transporter using a dipeptide library. Nat. Commun. 4:2502 doi: 10.1038/ncomms3502 (2013).